Character displacement of Cercopithecini primate visual signals Animal visual signals have the potential to act as an isolating barrier to prevent interbreeding of populations through a role in species recognition. Within communities of competing species, species recognition signals are predicted to undergo character displacement, becoming more visually distinctive from each other; however, this pattern has rarely been identified. Using computational face recognition algorithms to model primate face processing, we demonstrate that the face patterns of guenons (tribe: Cercopithecini) have evolved under selection to become more visually distinctive from those of other guenon species with whom they are sympatric. The relationship between the appearances of sympatric species suggests that distinguishing conspecifics from other guenon species has been a major driver of diversification in guenon face appearance. Visual signals that have undergone character displacement may have had an important role in the tribe’s radiation, keeping populations that became geographically separated reproductively isolated on secondary contact. Individuals from closely related species are often at risk of mating with each other and producing hybrids with reduced fitness. In addition to the reproductive disadvantages of interspecific matings, there may also be ecological advantages that favour mixing with individuals of the same species in tasks such as foraging [1] . Theory predicts that costly mismatings and associations with heterospecifics can be avoided by the evolution of species recognition signals that reliably identify individuals of the same species [2] , [3] . To improve discrimination between groups, species recognition signals are expected to undergo character displacement whereby phenotypic differences between two or more populations become accentuated where their ranges overlap [4] . Understanding the process of character displacement is particularly important because it has the potential to drive speciation events by creating new isolating barriers within a species that competes with different heterospecifics in different parts of its range [1] . Character displacement of visual signals has been demonstrated for single species and species pairs [5] , [6] , [7] ; however, there is very little evidence that this process has had an important and general role in larger lineages [8] , [9] , [10] . Comparative studies of character displacement in acoustic signals are more common, and while there are some clear examples of character displacement [11] , the opposite pattern of increased similarity between sympatric heterospecifics has also been identified [12] . These findings raise doubts about whether species recognition has had an important and widespread role in driving visual signal diversification and creating and maintaining reproductively isolated species. Here we investigate whether the colourful face patterns of guenon monkeys (tribe: Cercopithecini, Fig. 1 ) have appearances that show evidence of character displacement. This would be consistent with a role for face patterns in distinguishing conspecifics from heterospecifics. The guenons are a group of 25–36 primate species [13] , [14] that have radiated rapidly in the forests of Central and West Africa in the last 11 Ma. Many guenon species form mixed species associations with one another [15] , travelling and foraging together—behaviour that undoubtedly increases the likelihood of interspecific encounters that could have negative consequences for fitness such as hybrid matings. Captive matings and occasional reports of hybridization in the wild show that many, if not all, Cercopithecini species pairs have the potential to produce at least partially fertile hybrid offspring; however the overall rarity of hybrids in the wild suggests that selection against hybrids and reproductive interactions with heterospecifics is strong [16] . This led Kingdon [17] , [18] , [19] to propose that the diversity of guenon face patterns, along with other potential species recognition signals such as vocalizations [20] , [21] and species-specific movement patterns [18] , might be the result of character displacement between the signals of species at risk of hybridizing in order to promote reproductive isolation. 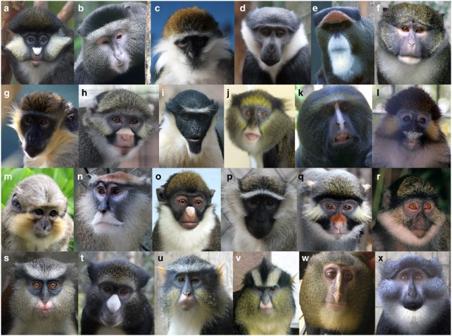Figure 1 Examples of guenon faces, illustrating interspecific diversity. Species: (a)Cercopithecus ascanius, (b)C. mitis, (c)Chlorocebus aethiops, (d)C. lhoesti, (e)C. neglectus, (f)Allenopithecus nigroviridis, (g)Ch. sabaeus, (h)C. sclateri, (i)C. diana, (j)C. campbelli, (k)C. hamlyni, (l)C. cephus, (m)Miopithecus talapoin, (n)Erythrocebus patas, (o)C. petaurista, (p)Ch. tantalus, (q)C. erythrotis, (r)C. erythrogaster, (s)C. mona, (t)C. nictitans, (u)C. wolfi, (v)C. pogonias, (w)C. lomamiensis, (x)C. preussi. (w) by M. Emetshu, reproduced with permission of K. Detwiler and J. Hart, (r) with permission of N. Rowe, all other images are by the author W. Allen. Figure 1 Examples of guenon faces, illustrating interspecific diversity. Species: ( a ) Cercopithecus ascanius , ( b ) C. mitis , ( c ) Chlorocebus aethiops , ( d ) C. lhoesti , ( e ) C. neglectus , ( f ) Allenopithecus nigroviridis , ( g ) Ch. sabaeus , ( h ) C. sclateri , ( i ) C. diana , ( j ) C. campbelli , ( k ) C. hamlyni , ( l ) C. cephus , ( m ) Miopithecus talapoin , ( n ) Erythrocebus patas , ( o ) C. petaurista , ( p ) Ch. tantalus , ( q ) C. erythrotis , ( r ) C. erythrogaster , ( s ) C. mona , ( t ) C. nictitans , ( u ) C. wolfi , ( v ) C. pogonias , ( w ) C. lomamiensis , ( x ) C. preussi . ( w ) by M. Emetshu, reproduced with permission of K. Detwiler and J. Hart, ( r ) with permission of N. Rowe, all other images are by the author W. Allen. Full size image Kingdon’s observational investigations using simple scoring measures such as the ratio of light-to-dark tones did not show any clear evidence for character displacement of face patterns, and his writing indicates frustration at the difficulty of quantifying such complex patterns [17] , [19] . Here we establish perceptually realistic measures of face pattern variation across the guenons from a new database of standardized digital photographs of frontal and profile views of 22 guenon species. To enable the colour, shape and pattern information contained within such complex patterns to be studied quantitatively, we apply the ‘eigenface’ technique [22] , [23] developed in the field of computer vision for machine recognition of human faces. The eigenface approach extracts the principal axes of variation in complex visual patterns in a way that is thought to be similar to how such patterns are encoded by the primate brain [24] , [25] . Eigenfaces can therefore be used to define a multidimensional face-space where geometric distances between objects provide a perceptually realistic and objective measure of visual distinctiveness known to correlate strongly with human assessment of human face visual distinctiveness [26] . While it is not yet known whether this measure also correlates highly with guenons’ judgements of visual distinctiveness, considering the known similarities between human and non-human primate face processing [27] , [28] , [29] , [30] , [31] and category discrimination mechanisms [32] , it seems likely. This computational approach also allows species recognition to be modelled as a machine classification task enabling identification of which species might be misclassified as another on the basis of visual appearance. We compare visual distinctiveness in face-space and classification rates between species pairs to measures of the degree of sympatry between species pairs [33] . Degree of sympatry is used as a quantitative geographic descriptor of the strength of the interspecific interactions that could potentially drive character displacement. We test two contrasting predictions arising from the character displacement hypothesis: (1) if visual signals function as species recognition signals that mediate interactions between species, the appearance of signals should become increasingly distinctive with increasing levels of sympatry between species, after controlling for the effects of shared ancestry [34] ; (2) Conversely, if ecological factors unrelated to interspecific interactions are of primary importance then allopatric species should be more divergent in appearance than sympatric species because their habitats are likely to be less similar [12] , [35] . We also evaluate a prediction arising from the theory of differential fusion that could also explain a pattern of character displacement. Under differential fusion, only species that evolve sufficiently distinctive mating signals in allopatry survive as reproductively isolated species on secondary contact with closely related taxa [36] . This theory makes the specific prediction that signal diversification is either a random event or the outcome of ecological adaptation, and so it predicts that the rate of change in face pattern diversification should be independent of lineage age [8] . However, if signals have diversified under selection to promote reproductive isolation or mediate interspecific interactions, we would expect the rate of change in phenotypes to be more rapid in younger lineages. Analyses show support for our first prediction that frontal views of guenon faces are more distinctive with increasing levels of sympatry between species, but against the differential fusion hypothesis as face pattern diversification is more rapid in younger lineages. The most likely interpretation of these findings is that guenon face patterns have evolved under selection to promote reproductive isolation in the tribe. Guenon eigenfaces captured visual distinctiveness The eigenface decomposition of the set of species mean faces successfully summarized and quantified variation in guenon face pattern appearance ( Fig. 2 , Supplementary Movie 1 ). Geometric distances between species in face-space conformed to human viewer expectations about the visual distinctiveness between pairs of species ( Fig. 3 ). 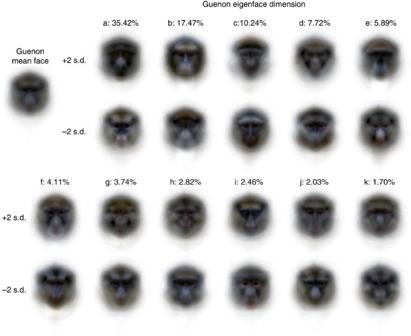Figure 2 The first 11 frontal eigenfaces. Eigenfaces are illustrated by reconstructing the faces produced by eigenface scores±two s.d.’s from the mean of the 22 species’ eigenface scores. Each dimension responds to features of guenon face patterns such as nose spots, eyebrow patches and beards of decreasing importance to overall variation in the set. For example, the first eigenface mainly describes how light or dark the face is and the second eigenface contrasts a light beard and dark eyebrow patch with dark cheeks and a yellowish eyebrow patch. More detailed and less common features were quantified by later components. Together, components 1 and 2 account for 52.89% of variance in estimates of guenon long, medium and short wavelength photoreceptor responses and the first 11 components describe 93.6% of variance. For the current application, the goal of achieving accurate reconstruction and recognition of new faces was more important than dimension reduction; we hence report the results of a guenon face-space based on all 21 eigenfaces. Figure 2 The first 11 frontal eigenfaces. Eigenfaces are illustrated by reconstructing the faces produced by eigenface scores±two s.d.’s from the mean of the 22 species’ eigenface scores. Each dimension responds to features of guenon face patterns such as nose spots, eyebrow patches and beards of decreasing importance to overall variation in the set. For example, the first eigenface mainly describes how light or dark the face is and the second eigenface contrasts a light beard and dark eyebrow patch with dark cheeks and a yellowish eyebrow patch. More detailed and less common features were quantified by later components. Together, components 1 and 2 account for 52.89% of variance in estimates of guenon long, medium and short wavelength photoreceptor responses and the first 11 components describe 93.6% of variance. For the current application, the goal of achieving accurate reconstruction and recognition of new faces was more important than dimension reduction; we hence report the results of a guenon face-space based on all 21 eigenfaces. 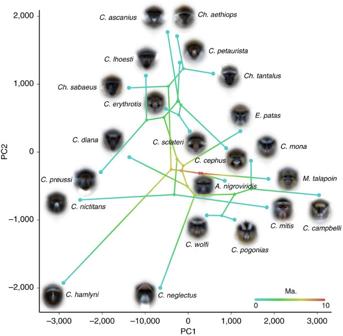Figure 3 Phylomorphospace of the first two eigenface dimensions. This shows the position of each species on the first two axes, giving an indication of the relative visual distinctiveness of species. Connections between points show species’ phylogenetic relationships38. Branch colour indicates distance from the root. Full size image Figure 3 Phylomorphospace of the first two eigenface dimensions. This shows the position of each species on the first two axes, giving an indication of the relative visual distinctiveness of species. Connections between points show species’ phylogenetic relationships [38] . Branch colour indicates distance from the root. Full size image Increased distinctiveness of frontal views in sympatry As we found mixed evidence for whether the face distinctiveness and sympatry measures contained phylogenetic signal ( Table 1 ), we tested for relationships between variables using both standard Mantel tests without phylogenetic correction and phylogenetically permuted (pp) partial Mantel tests [37] with a relatively weak phylogenetic correction ( k =2) [37] to assess whether findings were robust to different evolutionary models. We tested three different face pattern similarity metrics. The first two were the multivariate Euclidian distances in two different eigenface-space-derived models of face pattern learning, the mean face model and the exemplar model (Methods). The third was the recognition rate matrix between species from the species recognition classification task. These were compared with two spatial similarity metrics; degree of sympatry and geographic range overlap (Methods). All tests found support for the hypothesis that frontal facial distinctiveness and recognition performance were higher between species that had higher degrees of sympatry ( Table 2 ). All relationships were stronger for the geographic range overlap measure than the degree of sympatry geographic measure. Table 1 Phylogenetic signal in guenon eigenface scores. Full size table Table 2 Results of Mantel tests of association between frontal view face pattern matrices and geographic matrices. Full size table Profile views recognized more reliably in sympatry There was no relationship between either of the profile face pattern distinctiveness measures and the degree of sympatry, or geographic range overlap between species ( Table 3 ). However, the species recognition classification rate was significantly higher with increasing geographic range overlap, although not with increasing degree of sympatry. The significance of these relationships was not altered when different phylogenetic permutations were used for the Mantel tests. Table 3 Results of Mantel tests of association between profile view face pattern distinctiveness and species recognition classification matrices, and the geographic matrices. Full size table Diversification is more rapid in younger lineages In order to evaluate the differential fusion hypothesis, we measured the rate of change in the distinctiveness of face pattern scores between each node and an ancestral reconstruction of the face pattern of its direct ancestor, and examined how this was related to lineage age. We observed a strong negative correlation between the rate of change in face pattern distinctiveness and lineage age (using the Arnold et al. [38] tree, Pearson's r (40)=−0.413, P =0.0065, using the Guschanski et al. [39] tree, Pearson's r (40)=−0.483, P =0.0042) showing that the rate of change in face pattern appearance is more rapid on shorter branches. Phylogenetic signal in face pattern traits To understand the evolution of guenon face pattern traits and incorporate phylogenetic signal into analyses appropriately, we assessed relationships between guenon facial similarity and genetic similarity. We used Mantel tests to associate the face pattern distinctiveness measures with genetic distance between species pairs, taken as the square root of shared branch length. Across the whole tribe there was no significant relationship between the frontal similarity scores and genetic distances taken from either the Arnold et al. [38] tree (Mantel r (229)=0.0658, P =0.2829) or the Guschanski et al. [39] tree (Mantel r (229)=0.0752, P =0.1846). Correlations between the profile similarity scores and genetic distances approached significance (Arnold et al. [38] tree, Mantel r (229)=0.173, P =0.0613; Guschanski et al. [39] , Mantel r (229)=0.165, P =0.0728). However, when Allenopithecis nigroviridis and Miopithecus talapoin , the two species that diverged first in the guenon radiation and that also have faces with indistinctive appearances ( Fig. 3 ) were excluded, both frontal (Arnold et al. [38] tree, Mantel r (229)=0.241, P =0.006; Guschanski et al. [39] , Mantel r (229)=0.223, P =0.0093) and profile (Arnold et al. [38] tree, Mantel r (229)=0.198, P =0.0148; Guschanski et al. [39] , Mantel r (229)=0.184, P =0.0165) distinctiveness were significantly lower in more closely related species. We tested for phylogenetic signal in each guenon eigenface using Pagel’s λ [40] in the R package ‘caper’ [41] to investigate whether species’ scores on each of the eigenface dimensions evolve according to a Brownian motion model of phenotype change. The results show that, while some traits contain phylogenetic signal, others, especially the smaller eigenfaces dimensions, do not ( Table 1 ). This is fairly typical for mammalian coloration traits that frequently show a high degree of evolutionary lability, particularly in detailed aspects [42] . No spatial autocorrelation in guenon phylogeny As the guenon tribe has undergone repeated radiations across Central and West African forests, genetic distances between study species and geographic data are uncorrelated (Mantel tests: geographic range overlap and Arnold et al. [38] phylogenetic distance, Mantel r (229)=0.0409, P =0.2821; Guschanski et al. [39] , Mantel r (229)=0.0124, P =0.7545; degree sympatry and Arnold et al. [38] phylogenetic distance, Mantel r (229)=0.0167, P =0.6240; Guschanski et al. [39] , Mantel r (229)=0.0024, P =0.9811). Although speciation in the guenons is primarily allopatric [39] and no pairs of sister species are found in sympatry, over the tribe as a whole closely related species have neither particularly high nor low range overlap scores. Species classification from eigenface scores is reliable We modelled species recognition as a perceptual task by performing a computational simulation of a species identification task. Each of the original images was projected into the eigenface-space defined by the species average faces. A machine classifier made species identity decisions based on the minimum Euclidian distance between an original face’s scores and the average eigenface scores for a set of species. The correct species was identified in 94.16% of frontal views and 84.91% of profile views indicating that the signal could function effectively as a species recognition signal. The most common misclassifications were between closely related species with very similar appearance, for example, all the Ch. aethiops recognition errors were for Ch. sabaeus and 5.88% of C. erythrotis examples were classified as C. sclateri . Taken together, these results are consistent with the pattern of signalling phenotypes predicted by the process of character displacement driven by interspecific interactions between species [34] . This indicates a role for facial signals in communicating conspecific status [17] , [18] , [19] . To send their message reliably, species recognition signals should be easily discriminable from those of sympatric heterospecifics. As it is probable that guenons find it easier to recognize and remember faces as they become more distinctive [27] , [43] , improved identification and memorability provides a clear cognitive mechanism for how increased interspecific distinctiveness could mediate interactions between species. The relationship between face pattern distinctiveness and degree of sympatry was less clear-cut for profile views of faces than frontal views of faces. Evidence suggests that most interactions between guenons take place face-to-face [18] , and face recognition performance in humans is much better for frontal views [43] . As such, it is expected that the front of the face should be the main target of selection for improved species recognition. Given the evidence for low hybrid fitness in the Cercopithecini [16] , we suggest that the pattern of character displacement is most consistent with the process of reinforcement of signal phenotypes to strengthen reproductive isolation between species [36] . Under this hypothesis, phenotypes diverge because they are under positive selection when each population shows assortative mating because either hybrids have lower fitness or interspecific matings are costly. Although further work will be required to confirm reinforcement, the process is highly plausible. Range shifts brought on by expansions and contractions in African forest cover will have brought populations of guenons from different parts of each species’ range into contact with heterospecific guenon competitors with different appearances [33] . The composition of heterospecifics’ signals creates new selective environments causing signals used in mate choice to undergo character displacement and diverge, strengthening mating barriers between the two populations when they come into contact. This could potentially lead to the formation of new species if isolating barriers reduce gene flow sufficiently [2] . Thus, guenon face patterns may be ‘speciation phenotypes’ [44] , traits whose divergence contributes to reduced gene flow during speciation. Interspecific competition between species unrelated to reproduction may also have had an important influence on creating the observed pattern of character displacement [1] . Indeed, this is suggested by the lack of sexual dichromatism in the faces of the majority of guenon species, a common property of signals not used in mating behaviour [45] . Character displacement may support social ecological interactions between conspecifics such as identification of foraging partners and reduced costs of interspecific aggression. The pattern of character displacement could also be occurring without any direct interspecific interactions under the ‘noisy neighbours’ model where the signals of sympatric heterospecific guenons can interfere with and mask conspecific signals, resulting in selection for distinctive patterns [46] . However, given that we know guenons occasionally do hybridize, and because visual signals have relatively limited ranges (unlike acoustic signals), we suggest that, while noise may contribute to divergence, overall this process is unlikely to be of major importance. Our results also suggest that other alternative explanations for the pattern of increased distinctiveness in sympatry that are not based on interactions between species are unlikely [36] . The faster rate of change in face pattern distinctiveness on shorter lineages argues against differential fusion explaining the association because this process predicts novelty arising independently of lineage age [8] . We found that the face patterns of younger lineages change faster, suggesting that diversification is most rapid at the time of speciation events. This finding is consistent with the hypothesis that guenon face patterns contribute to reproductive isolation in the early stages of speciation. The idea that runaway sexual selection could explain guenon face patterns is also implausible, given that we know initial divergence in guenons mainly occurs in allopatry [39] . There was no support for our alternative prediction that if ecological factors unrelated to interspecific interactions were of primary importance in driving the diversification of guenon face patterns, then greater similarity in signal appearance with increasing levels of sympatry would be expected. Although we do not discount the likely effect of lighting environment on particular aspects of signal appearance, such as colours being selected for camouflage or conspicuousness against typical backgrounds [47] , our results show that the appearance of sympatric species is an important driver of diversification in overall appearance of guenon multicomponent signals. Our results contrast with a recent comparative study of Amazonian bird song that found greater similarity of acoustic properties in sympatry than that expected by chance [12] . Clearly character displacement of the signals of closely related species is neither ubiquitous or extremely uncommon [8] , [10] . Identifying the conditions that promote either clustering or displacement of signals within communities of competing species is an important next step. Our results also contrast somewhat with those of a recent study that found an association between face pattern complexity and the number of sympatric species across all catarrhines [48] . Although the aims of the studies are different, the apparent difference in results is likely to be due to the measures used; both pattern complexity and the overall number of sympatric species may not be well suited to identify and measure character displacement. The perceptual parameter under selection when signals are undergoing character displacement is distinctiveness , specifically between those species that interact. Many primate species have appearances that are not complex, yet remain highly visually distinct—an example is the bald bright red face of the Uakari ( Cacajao calvus ), which is extremely simple yet highly distinctive and completely different to the face of any species it is sympatric with. Similarly, what matters for signal form is not necessarily the total number of sympatric species but the appearance of those sympatric species. The total number of sympatric species is perhaps not important until it becomes difficult to find an empty area of face-space. Given that large areas of face-space and novel design opportunities remain unused in the guenons ( Fig. 3 ), this seems unlikely to be a constraint at present for the tribe, although the ability to occupy new face-space may be limited by genetic, developmental or mechanistic constraints on the evolution of certain phenotypes [42] or by fitness valleys that must be circumvented. Guenons appear to evolve increased distinctiveness by acquiring or losing traits found on several species such as nose spots or eyebrow patches, or by elaborating on existing traits evolving new patch colours or shapes. Overall, the relationships observed between face patterns and sympatry patterns observed, although statistically significant, are relatively weak (low r ). Partly, this is related to unavoidable noise that is introduced when making detailed face pattern measurements, but mainly because, while there may be selection for increased distinctiveness in sympatry, there is not necessarily selection for increased similarity in allopatry. We also emphasize that there are many other factors we were unable to consider in this study that may contribute to both the appearance of each species’ face patterns and the likelihood of interactions between species, such as habitat use, typical group sizes and the propensity for species to form polyspecific associations [18] . Correlations with distinctiveness measures were consistently stronger for the geographic range overlap measure compared with the degree of sympatry measure. Geographic range overlap is relatively higher than degree of sympatry when one species in a pair has a very small range that is entirely within the range of a species with a large range. Thus, this pattern may be best explained by selection for species with small ranges to evolve particularly distinctive patterns on the periphery of face-space, whereas species with larger ranges that contact many other species occupy more central regions. In summary, we have shown that in a large tribe of primates, face patterns have evolved to be especially distinctive from those that they share more of their range with. The likely cause of this relationship is that face patterns function as species recognition signals to promote and maintain reproductive isolation between species through either ecological or reproductive character displacement. The observed pattern is likely the result of the process of reinforcement, a key mechanism that can create new species [2] . In demonstrating this in our own Order, we open the question of the role of visual recognition in the evolution of our own lineage. Data collection We took digital images of Cercopithecini primates held in captivity in US and UK zoos and a wildlife sanctuary in Nigeria (CERCOPAN) using a calibrated camera set-up to enable estimation of guenon cone photoreceptor catches and subject illumination [49] . This also allowed the photographer to have control over scene capture and lighting conditions, while our modelling procedures allow us to investigate colours in images irrespective of the lighting conditions under which they were taken. Collecting high-quality image data for wild guenons would have been close-to-impossible because of their rarity, dense habitats and arboreality. We used a Canon T2i fitted with Canon EF-S lenses of either 18–55, 55–250 or 75–300 mm depending on conditions. A circular polarizing filter was fitted to reduce specular highlights off hair and glass. To photograph moving subjects we minimized exposure times by using a wide aperture (typically f/5.6) and high ISO rating (typically ISO 800). We collected multiple in-focus images of each individual subject in frontal and profile body positions (within 10° of ideal) under indirect light (that is, overcast conditions outdoors or diffuse artificial light indoors). We avoided images containing objects that occluded a portion of the subject’s face, those where the subject had a non-neutral facial expression, and repetitions of the subject in the same body position. We made sure to exclude all potential captive hybrids by using zoo records and information from the Old World Monkey Taxon Advisory Group. In addition to these sources, guenon hybrids usually exhibit phenotypic visual traits of both parent species, providing a final visual confirmation of the absence of hybridization. Our analysis included 719 frontal and 698 profile images of 149 individuals from 22 Cercopithecini species (following Groves [13] ): A. nigroviridis (6M, 5F), Cercopithecus ascanius (5, 7), C. campbelli (1, 1), C. cephus (1, 2), C. diana (6, 5), C. erythrotis (2, 2), C. hamlyni (1, 1), C. lhoesti (3, 2), C. mitis (1, 2), C. mona (12, 10), C. neglectus (2, 4), C. nictitans (8, 15), C. petaurista (3, 4), C. pogonias (1, 0), C. wolfi (3, 4), C sclateri (4, 4); Chlorocebus aethiops (2, 0), Ch. sabaeus (3, 1), Ch. tantalus (2, 2); Erythrocebus patas (2, 2); M. talapoin (3, 2). Although both Grubb et al. [14] and Groves [13] identify C. diana and C. roloway as separate species, and we were able to photograph one male and one female C. roloway , we combined data for these former subspecies on the basis of their observed visual similarity and because both species are sympatric with the same species ( C. campbelli, C. nictitans, C. petaurista and Ch. sabaeus ) in order to avoid exaggerating similarities and differences in distinctiveness between species. Incomplete taxon sampling has the potential to affect results if missing taxa form a non-random and influential set. Our sample is likely to have minimal bias—we sampled all the species known to be held in captivity in the United States, United Kingdom and Nigeria. This includes all of the most common and wide-ranging Cercopithecini species. Of the species not included, the majority have only recently been raised to the species level, have limited ranges or are rare in the wild. They are as follows: Cercopithecus albogularis (former C. mitis subspecies), C. denti (not in captivity, rare, former C. pogonias subspecies with similar appearance), C. dogetti (not in captivity, rare, former C. mitis subspecies with similar appearance), C. dryas (not in captivity, rare), C. erythrogaster (not in captivity, rare), C. kandti (not in captivity, rare, former C. mitis subspecies with similar appearance and limited range), C. lomamiensis (not in captivity, rare, only recently identified), C. lowei (not in captivity, rare, former C. campbelli subspecies with similar appearance), C. solatus (not in captivity, rare, limited range), Chlorocebus cynosuros (not in captivity, Ch. aethiops former subspecies), Ch. djamdjamensis (not sympatric with any study species, not in captivity, rare, former Ch. aethiops subspecies) and Miopithecus ogouensis (not in captivity, former M. talapoin subspecies). Former subspecies generally have similar appearances to the sister species we sampled. By joining the ranges of former subspecies together we take a conservative approach to test whether face pattern distinctiveness increases in sympatry. Image processing Images were collected in RAW format and converted to linearized TIFFs using DCRAW [50] . We modelled the retinal responses of a guenon receiver to the visual scene recorded by the camera. To do this we required pixel values to be proportional to photon counts and so removed a slight remaining nonlinearity in sensor response to light intensity using a polynomial transform [49] . We then converted sensor RGB responses from the camera’s colour space to guenon LMS (long, medium and short wavelength cone photoreceptor) colour space. We estimated the camera’s spectral sensitivity empirically by imaging a reflectance standard through narrow band-pass filters and comparing camera responses and spectrometer readings. In conjunction with image exposure settings and estimates of Cercopithecus photoreceptor sensitivity [5] , [51] , [52] , we used standard colour [52] space transformation methods [49] , [53] , [54] to calculate the matrix transform between the camera and guenon colour space. To correct for differences in ambient light and photographic exposure, and to model colour constancy processes in mammalian colour vision, we rescaled each channel with respect to an estimate of the white point. As good practice is to care for captive primates ‘hands-off’ without any direct human contact, and because lighting was sometimes different inside and outside of enclosures, we were unable to always measure a reference standard under exactly the same illuminant as the subject. Instead, we applied a computational colour constancy algorithm to images [55] . First, we cropped the subject out from areas of the background that either emitted light or were clipped above the dynamic range of the camera (typically the sky, artificial lights and specular reflections) and those that were under obviously difference illumination from the subject (for example, an artificially lit area outside a naturally lit enclosure). To correct for the colour of the illuminant we then made the grey world assumption [56] that the average colour of surfaces in a scene is grey, by equalizing the cone responses at each pixel based on the ratios of average long (L), medium (M) and short (S) wavelength photoreceptor responses. We then identified the most reflective surface in the scene (that is, the maximum of all L, M and S values) and set this value as the white point, scaling other values accordingly. This perfect reflectance test assumes that there is a surface in the scene that reflects all light at a wavelength that one cone class is most sensitive to. We compared these white point estimates to measurements of the white patch on a Macbeth ColorChecker chart for images in which we considered there was good correspondence between the incident illumination of the subject and reflectance standard. We found a mean difference of 8.56% between the estimates and physical white points. This compares well with the mean 9.14% white point difference we have recorded between different images of the same physical standard taken in short succession from similar viewpoints under natural illumination [57] . Our next step was to segment out each individual’s head from the background. To do this we used a semi-automated outlining programme in MATLAB, which uses spline interpolation to connect points selected by the user on the outline of the head. For frontal images, we selected the region bounded by the tips of hair originating along the jawline, around the outside of ears and over the top of the head. For profile images, we selected the region bounded by the tips of hair originating along an estimate of the coronal plane, cutting straight across the neck at the base of the jaw. We standardized these cropped faces for size, orientation and position by transforming two landmarks to fixed coordinates using bilinear interpolation. For frontal images, we chose the outside corner of each eye as landmarks. For profile images, we flipped images so that they were all facing left and used the outside corner of the eye and the opening of the ear as landmarks. Images were then all trimmed to the same size. We calculated the average LMS colour of all images and set this as the background colour. Partly to remove noisy pixels from the image caused by high ISO settings, but more importantly to standardize the texture of the hair across images by normalizing the effect of camera shake, we applied a circular averaging filter of a diameter that gave a perceptually validated blur metric [58] score of 0.75, resulting in a set of equally slightly blurred images. We then determined the mean frontal and profile face of each individual, the species mean face from all individual average faces and the guenon mean face from all species average faces. We pooled both male and female faces in determining the species average faces as a series of discriminant factor analyses did not find significant differences between males and females for any of the study species that could be used to reliably classify and distinguish the sexes on the basis of face pattern appearance. Calculating facial distinctiveness We calculated eigenfaces from two alternative models of guenon face learning. The mean face model implicitly assumes that guenons code different species’ face patterns as the average of all examples encountered by calculating eigenfaces from the species average face images. The alternative exemplar model assumes that the face pattern of each different species is coded by examples that fit that category; in this case we construct eigenfaces based on five randomly selected example images of each species from the entire frontal or profile sets. Both the mean face and exemplar models produced very similar eigenface and distinctiveness scores. In both models, images were first resized to 98 × 75 × 3 pixels due to processing limitations. LMS responses were concatenated into a single vector for each image and the guenon average face vector was subtracted before performing PCA on the matrix of mean-shifted image vectors. Interspecific visual distinctiveness was then scored as the mean of the multivariate Euclidian distances between component scores for all species–species pairs. We determined eigenfaces using both standard PCA and phylogenetic PCA (pPCA) [59] for the eigenface decomposition. Phylogenetic PCA incorporates the evolutionary relationships between species to control for expected phylogenetic covariance in data to result in components that describe the axes of non-phylogenetic variation. The two methods will therefore find major axes that differ most in orientation when there is strong phylogenetic signal in face pattern appearance. Here we report only the results of non-phylogenetic PCA because if all dimensions of the space are used, variance is conserved so that the multidimensional distance between species (on which our distinctiveness measure is based) is identical in PCA space and pPCA space [60] . We confirmed this by running tests on measures derived from the pPCA space and found the same pattern of results. Species’ scores on each dimension are also uncorrelated in PCA space, whereas this is not necessarily the case in pPCA space. For our purpose this makes visualization and interpretation of the data more straightforward. As we do not perform tests on components that assume they are independent of phylogeny, this advantage of pPCA is not relevant. As our objective was to achieve accurate reconstruction and recognition of new faces rather than dimension reduction, we report the results of a guenon face-space based on all 21 eigenfaces. An animation showing the reconstruction of species mean faces from their eigenface scores is available ( Supplementary Movie 1 ). Guenon phylogenetics While the traditional taxonomic breakdown of the Cercopithecini into the present genus and superspecies groups has remained relatively stable in recent decades, the inferred phylogenetic relationships between Cercopithecini species within and between superspecies groups have been under flux [61] , [62] , [63] , [64] . However, recent studies using multiple sequences have produced well-resolved phylogenies with fairly consistent topologies. In order to establish whether results are sensitive to differences in tree topology and divergence dates found by recent molecular phylogenies of the guenons, we repeated all our phylogenetic analyses using the consensus trees of both Arnold et al. [38] and Guschanski et al. [39] ( Fig. 4 ). Both these trees use multiple molecular sequences and result in well-supported fully resolved consensus trees. Guschanski et al. [39] analyse only the mitochondrial genome, whereas Arnold et al. [38] analyse both mitochondrial and nuclear gene sequences. We utilized both trees because there are some discrepancies, likely to be due to incomplete lineage sorting and hybridizations. Notably in the mtDNA-only tree [39] , C. hamlyni is sister to the Ch. aethiops group rather than C. neglectus ; the C. lhoesti group is sister to the C. cephus group rather than the Ch. aethiops group; and E. patas diverges from the ancestor to the C. mitis , C. cephus and C. lhoesti groups rather than being sister to C. lhoesti in the nuclear+mtDNA tree [38] . In Arnold et al. [38] , which analysed multiple individuals of many species, the individual samples for C. cephus , C. mona, C. nictitans and Ch. tantalus were not monophyletic in the consensus tree. We resolved this by selecting the clade with the highest number of individuals. C. sclateri was not included in either tree, so we inserted it as sister to C. erythrotis with the divergence date half-way along the branch as C. sclateri was formerly considered a subspecies of C. erythrotis [13] , [14] . 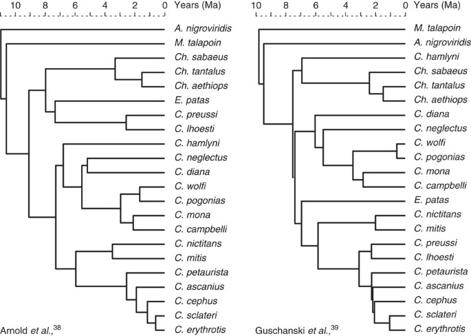Figure 4 The two consensus phylogenetic trees of the Cercopithecini study species used for phylogenetic analyses38,39. Figure 4 The two consensus phylogenetic trees of the Cercopithecini study species used for phylogenetic analyses [38] , [39] . Full size image Measuring degree of sympatry We obtained range maps as shapefiles for all Cercopithecini species from the International Union for Conservation of Nature (IUCN). For all the taxa that we were unable to photograph where there is debate over whether they are species or subspecies [13] , [14] , we combined the range with the full species that we were able to photograph. This meant that the C. mitis range includes that of C. albogularis , C. dogetti and C. kandti , the C. pogonias range included C. denti , C. campbelli included C. lowei , Ch. aethiops included Ch. pygerythrus and Ch. cynosuros and the M. talapoin range included M. ogouensis. Although there are some variations in visual appearance in these groups, this approach was considered preferable to the errors in measuring degree of sympatry that would result from excluding these areas. Although recent anthropogenic forces have influenced the amount of suitable habitat available to guenons, this has largely resulted in habitat fragmentation rather than a reduction or shift in limits of geographic ranges as recorded in range maps. We measured the degree of sympatry as the area of range overlap divided by the total area of the combined ranges of both species [33] . We also measured habitat range overlap as the area of overlap divided by the area of the taxon with the smaller range. This measure will give higher scores to pairs where one species is found entirely within the range of another, even if the other is widely distributed. It thus attaches more weight to the impact of wide-ranging species on species with smaller ranges. These factors were calculated for each sister species dyad (total=231) using the Mapping Toolbox in MATLAB. Statistical analysis To assess the relationship between degree of sympatry and facial pattern distinctiveness, we conducted Mantel tests and phylogenetically permuted (pp) partial Mantel tests [37] , [65] , [66] , the appropriate tests for data expressed as pairwise distances between taxa [67] . This test calculates the Z statistic for the observed facial similarity and degree of sympatry distance matrices F and S : The analysis compares Z with the expected null distribution when distance matrices are uncorrelated. This is calculated by permuting rows and columns of one of the matrices, holding those of the other fixed, recalculating Z , and repeating this a large number of times. For phylogenetically permuted tests, permutations between taxa are made dependent on their relatedness, with more closely related taxa being switched more frequently in order to account for the phylogenetic dependence of data points [37] . The tests reported are based on 10,000 permutations. Concerns have been raised about the poor statistical performance of partial Mantel tests, including low power and inflated type-1 error rates under some circumstances [68] . However, the phylogenetic permutation method has been shown to deal successfully with the issues and to our knowledge, phylogenetically permuted Mantel tests are the only current way to test hypotheses regarding relationships between variables that can only be expressed as distance matrices and that might exhibit autocorrelation due to phylogenetic dependence [67] , [69] . Species recognition from guenon eigenfaces To investigate whether an eigenface model can successfully recognize species status in our data, we undertook a computational recognition task. First, we projected the 719 frontal and 698 profile original images into the 21-dimension face-space to obtain eigenface scores for each image. The recognition algorithm determined identity as the minimum of the multivariate Euclidian distances between an original image’s scores and the set of species’ average scores. We then calculated the percentage correct classification rate for each species and the misclassification rate between each heterospecific species pair in order to evaluate how reliably images could be classified as the correct identity. When performing Mantel tests on recognition rates we analysed the log(misrecognition rate+1) to correct for the zero-biased and skewed distribution. Rate of face pattern diversification To examine how rapidly face patterns have changed in different lineages we used functions in the phytools package [70] to estimate the maximum likelihood ancestral eigenface scores at each node of both trees. We then calculated the change in distinctiveness between each ancestral node and its two descendants as the multivariate Euclidian distance between eigenface scores. The rate of change was the change in distinctiveness divided by the branch length. How to cite this article: Allen, W. L. et al. Character displacement of Cercopithecini primate visual signals. Nat. Commun. 5:4266 doi: 10.1038/ncomms5266 (2014).